HEB associates with PRC2 and SMAD2/3 to regulate developmental fates In embryonic stem cells, extracellular signals are required to derepress developmental promoters to drive lineage specification, but the proteins involved in connecting extrinsic cues to relaxation of chromatin remain unknown. We demonstrate that the helix-loop-helix (HLH) protein, HEB, directly associates with the Polycomb repressive complex 2 (PRC2) at a subset of developmental promoters, including at genes involved in mesoderm and endoderm specification and at the Hox and Fox gene families. While we show that depletion of HEB does not affect mouse ESCs, it does cause premature differentiation after exposure to Activin. Further, we find that HEB deposition at developmental promoters is dependent upon PRC2 and independent of Nodal, whereas HEB association with SMAD2/3 elements is dependent of Nodal, but independent of PRC2. We suggest that HEB is a fundamental link between Nodal signalling, the derepression of a specific class of poised promoters during differentiation, and lineage specification in mouse ESCs. Cooperation between epigenetic machinery and cellular signalling pathways occurs to drive specific cell fates. Within the early embryo and in embryonic stem cells (ESCs), the well-studied repression enacted by Polycomb repressive complex 2 (PRC2) at developmental promoters must be alleviated by exposure to extrinsic signals to drive differentiation [1] , [2] , [3] , [4] . PRC2 occupies most developmental promoters in ESCs, including those associated with transcription factors that drive differentiation towards neural, endodermal, mesodermal and trophectodermal fates [5] , [6] , [7] . How particular promoters become derepressed in response to extrinsic signals to cause a specific lineage to be formed is unknown, although a few examples have been described. During myoblast differentiation, MSX1 physically interacts with EZH2, one of the core components of PRC2, causing EZH2 to move away from repressed chromatin and toward the nuclear periphery [8] . Furthermore, the neurodevelopmental regulator, Geminin, directly inhibits Hox gene function by association with PRC2 within the neural tube [9] . These findings illustrate that coordination between the signals that drive differentiation and the derepression caused by PRC2 exists in different cellular contexts, but the molecular components that control the process in pluripotent stem cells are undefined. PRC2 and its associated function are highly conserved among animals [10] . The proteins that comprise this complex were originally identified as the Polycomb group (PcG) proteins in Drosophila where they function during body segmentation by selectively repressing the homeobox genes of the Hox cluster [11] , [12] , [13] . The function of PcG proteins as repressors of developmental genes is conserved in mammals, where they are found in multiprotein Polycomb repressive complexes, PRC1 and PRC2 (ref. 14 ). PRC2, containing EED, EZH2 and SUZ12, catalyses di- and trimethylation of lysine 27 on histone H3 (H3K27me2/3), which is an epigenetic mark that represses chromatin [2] , [15] , [16] , [17] , [18] . PRC2 is also critical for the creation of bivalent domains in ESCs. Bivalent domains are tagged by H3K27me3 and H3K4me3, and mark developmental promoters which are inactive in the undifferentiated state but are poised for rapid activation during differentiation [19] , [20] , [21] , [22] . In the mouse, PRC2 has a critical role in specifying lineage fates, leading to the hypothesis that it regulates the transition from pluripotency to differentiated states. In the mouse embryo, each PRC2 component is necessary for gastrulation, demonstrating an important in vivo role for PRC2 in lineage determination [7] , [23] , [24] , [25] , [26] . Likewise, in mouse ESCs, while these proteins are not essential for pluripotency, EED, SUZ12 and EZH2 are necessary for appropriate lineage specification, strongly suggesting that PRC2 is a general regulator of the transition from pluripotency toward more specific cellular fates [7] , [23] , [24] . Nodal signalling is essential for mesoderm and endoderm development [27] . The pathway utilizes serine threonine kinase receptors to phosphorylate intracellular proteins, SMAD2 and SMAD3 (refs 27 , 28 , 29 ). These proteins translocate to the nucleus and drive gene expression that is necessary for mesoderm and endoderm formation. Recently, SMAD2/3 was found to recruit the histone demethylase JMJD3 to the Nodal promoter in mouse ESCs, inducing the loss of the H3K27me3 and leading to Nodal transcription [30] , [31] . Thus, the SMAD2/3–JMJD3 complex relieves PRC2-mediated repression by altering chromatin conformation at the Nodal locus. It is unclear, however, whether this mechanism acts at mesodermal gene promoters genome-wide and whether the Nodal signalling pathway interacts directly with PRC2 to influence fate decisions. We have previously shown that the helix-loop-helix (HLH) proteins HEB and E2A are components of Nodal signalling in both human ESCs and the frog, Xenopus [32] . These proteins bind SMAD2/3, function as SMAD2/3 cofactors and are critical for Nodal signalling. In our current study, we find evidence that HEB functions with SMAD2/3 at distal enhancer elements and also directly associates with PRC2 at a subset of developmental promoters that are important for mesoderm and endoderm (ME) formation. In addition, we present functional experiments in mouse ESCs showing that HEB depletion results in ectopic and premature mesoderm and endoderm formation after the onset of differentiation. Our data strongly suggest that HEB/PRC2 marks a subset of lineage-specific bivalent promoters, and that HEB is essential for repression of loci that are necessary for mesoderm or endoderm formation. HEB occupies bivalent domains To examine where SMAD2/3 and its cofactor HEB bind chromatin in the genome of mouse ESCs, we performed chromatin immunoprecipitation (ChIP)-seq [33] using anti-SMAD2/3 and anti-HEB antibodies. 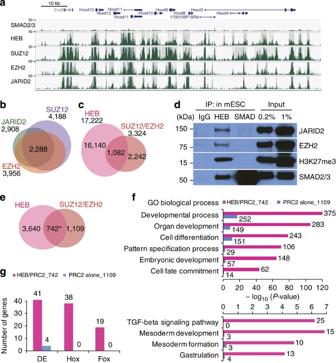Figure 1: HEB interacts with PRC2. (a) Genome browser representation of SMAD2/3, HEB, SUZ12, EZH2 and JARID2 binding patterns at theHoxdgene cluster in mouse ESCs. (b) Venn diagram comparing regions that associate with JARID2, SUZ12 and EZH2. (c) Venn diagram comparing regions that associate with HEB and both SUZ12 and EZH2. (d) Immunoprecipitation (IP) of HEB and SMAD2/3 (SMAD) in mouse ESCs. ESC lysates were used to pull down interacting proteins using anti-HEB and anti-SMAD2/3 antibodies. Western blot analysis shows that JARID2, EZH2, H3K27me3 and SMAD2/3 were immunoprecipitated with pulled-down complexes. Rabbit IgG was used as a negative control for IP. Input lysates were used as positive controls. (e) Venn diagram comparing the overlap of genes that neighbour either HEB-bound regions or both SUZ12/EZH2 bound regions within 10 kb from a TSS. Significance was tested using Fisher’s exact test (*P=1.19E-122). (f) DAVID GO analysis using the 742 genes neighbouring regions bound by HEB, SUZ12 and EZH2 (HEB/PRC2; pink) and the 1,109 genes neighbouring regions bound by SUZ12 and EZH2, but not HEB (PRC2 alone; blue). The number in the right end of each bar represents the number of enriched genes in each category. (g) Hand curated using definitive endoderm (DE) gene lists36,37and GO annotations forHoxandFoxgenes for the gene set containing both HEB and PRC2 (SUZ12 and EZH2) bound promoters (HEB/PRC2_742 genes) or PRC alone (PRC2 alone_1109 genes). We find that SMAD2/3 and HEB occupy 4,111 and 17,222 regions genome-wide, respectively (see Supplementary Table 1 for read counts and peak calls). When we examine HEB-bound regions, we find that ~29% (4,954 regions) and 40% (6,906 regions) of binding occurs within 5 and 10 kb, respectively, of a transcription start site (TSS: Supplementary Fig. 1a ). A close inspection of HEB occupancy at these regions using GREAT [34] , a programme that predicts the function of cis-regulatory elements, reveals broad domains covering the promoters of genes that are significantly enriched for developmental processes (Binom raw, P <1.0E-320), including the Hoxd gene cluster ( Fig. 1a ). Surprisingly, we find no evidence of SMAD2/3 binding at these loci. Figure 1: HEB interacts with PRC2. ( a ) Genome browser representation of SMAD2/3, HEB, SUZ12, EZH2 and JARID2 binding patterns at the Hoxd gene cluster in mouse ESCs. ( b ) Venn diagram comparing regions that associate with JARID2, SUZ12 and EZH2. ( c ) Venn diagram comparing regions that associate with HEB and both SUZ12 and EZH2. ( d ) Immunoprecipitation (IP) of HEB and SMAD2/3 (SMAD) in mouse ESCs. ESC lysates were used to pull down interacting proteins using anti-HEB and anti-SMAD2/3 antibodies. Western blot analysis shows that JARID2, EZH2, H3K27me3 and SMAD2/3 were immunoprecipitated with pulled-down complexes. Rabbit IgG was used as a negative control for IP. Input lysates were used as positive controls. ( e ) Venn diagram comparing the overlap of genes that neighbour either HEB-bound regions or both SUZ12/EZH2 bound regions within 10 kb from a TSS. Significance was tested using Fisher’s exact test (* P =1.19E-122). ( f ) DAVID GO analysis using the 742 genes neighbouring regions bound by HEB, SUZ12 and EZH2 (HEB/PRC2; pink) and the 1,109 genes neighbouring regions bound by SUZ12 and EZH2, but not HEB (PRC2 alone; blue). The number in the right end of each bar represents the number of enriched genes in each category. ( g ) Hand curated using definitive endoderm (DE) gene lists [36] , [37] and GO annotations for Hox and Fox genes for the gene set containing both HEB and PRC2 (SUZ12 and EZH2) bound promoters (HEB/PRC2_742 genes) or PRC alone (PRC2 alone_1109 genes). Full size image The broad domain of HEB at promoters and the strong enrichment of developmental processes are reminiscent of the bivalent domain signature observed at developmental promoters in mouse ESCs [19] , [21] . Therefore, we compared the genes which are adjacent to an HEB-bound element with the genes that contain bivalent domains in mouse ESCs ChIP-seq data [19] . We found that 32% (852/2,688) of the annotated bivalent promoters were occupied by HEB, suggesting that HEB marks a subset of poised developmental promoters in ESCs ( Supplementary Fig. 1b,c ). HEB associates with PRC2 at developmental promoters Since PRC2 is essential for the creation of bivalent domains and its components bind adjacent to developmental promoters in mouse ESCs [6] , [7] , we examined whether HEB interacts with PRC2. We compared the HEB-bound domains with the genome-wide occupancy of SUZ12, EZH2 and JARID2, which we obtained from published ChIP-seq data sets [35] ( Fig. 1a ). We identified 2,288 regions co-bound by EZH2, SUZ12 and JARID2 genome-wide ( Fig. 1b ). Then, we compared our HEB ChIP-seq data set with regions co-bound by EZH2 and SUZ12, and identified 1,082 regions that contain all three proteins ( Fig. 1c ). Overall, approximately one-third of the promoters bound by PRC2 are also bound by HEB. The overlap of SUZ12, EZH2, JARID2 and HEB at promoters is remarkable and suggests that HEB may bind directly to PRC2. Therefore, we examined whether HEB interacts with EZH2, JARID2 and H3K27me3. Immunoprecipitation of proteins from ESCs using anti-HEB and anti-SMAD2/3 antibodies, followed by western blotting with anti-JARID2, anti-EZH2, anti-H3K27me3 and anti-SMAD2/3 antibodies, showed that HEB associates with EZH2, JARID2, and H3K27me3 ( Fig. 1d ). Confirming our previous data in human ESCs, we found that SMAD2/3 interacts with HEB, but intriguingly, it does not associate with either EZH2 or JARID2. Thus, our data suggest that HEB associates directly with PRC2 and H3K27me3 at many developmental promoters. HEB/PRC2-bound promoters are enriched for ME regulators To examine whether HEB conferred function to PRC2-bound genes, we compared the genes whose promoters are bound by both HEB and PRC2 (HEB/PRC2) and those bound by PRC2, but not HEB (PRC2 alone). We identified 742 genes that contain promoter regions occupied by HEB, SUZ12 and EZH2 (HEB/PRC2) and 1,109 genes that contain promoter regions occupied by SUZ12 and EZH2, but not HEB (PRC2 alone, Fig. 1e ). Among the 742 HEB/PRC2-bound genes, 572 (77%) contain a bivalent domain ( Supplementary Fig. 1d ). To examine the function of genes containing promoters with either HEB/PRC2 or PRC2 alone, we performed DAVID Gene Ontology (GO) analysis (DAVID v6.7, http://david.abcc.ncifcrf.gov ) on these two gene lists and found that both groups have annotations significant for developmental process (HEB/PRC2, P =6.92E-120; PRC2 alone, P =6.31E-18; Fig. 1f ). Most intriguingly, those genes whose promoters are bound by HEB/PRC2 are enriched for terms that involve the TGF-beta signalling pathway ( P =6.28E-7), mesoderm development ( P =1.43E-7), pattern specification ( P =4.94E-71) and gastrulation ( P =6.90E-5). These terms were not enriched in the list of genes that were bound by PRC2 alone. Significance of DAVID GO term was shown with EASE score, a modified Fisher’s exact P -value. 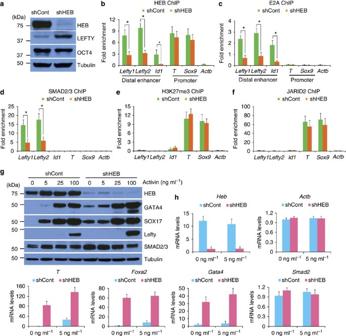Figure 2: Depletion of HEB drives ME differentiation. (a) Western blot analysis on control shRNA (shCont) and shHEB-treated mouse ESCs detected the protein expression of HEB, LEFTY and OCT4. TUBULIN was used for loading control. (b–f) Chromatin immunoprecipitation (ChIP) using anti-HEB (b), E2A (c), SMAD2/3 (d), H3K27me3 (e) and JARID2 (f) antibodies in either shCont (green) or shHEB (orange) ESCs. Pulled-down chromatin was analysed by qPCR using primers surrounding distal enhancer regions ofLefty1,Lefty2andId1and proximal promoter regions ofBrachyury(T) andSox9, which are occupied by PRC2 in mouse ESCs. TheActblocus was used as a negative control. Error bars are based on the s.d. derived from triplicate qPCR reactions and enrichment is calculated relative to input. *P<0.05 by Student’s pairedt-test with a two-tailed distribution. (g) Western analysis of HEB, GATA4, SOX17, LEFTY and SMAD2/3 in EBs after 4 days of differentiation from shCont or shHEB ESCs at different concentrations of Activin (0–100 ng ml−1) treatment. TUBULIN was used as a loading control. (h) qPCR with reverse transcription analysis of 4-day EBs derived from shCont (blue) or shHEB (pink) ESCs either without Activin (0 ng ml−1) or a low dose of Activin (5 ng ml−1). Expression was normalized toGapdhtranscript levels. Error bars represent s.d. calculated from triplicate qPCR reactions. Genes in each annotation category are listed in Supplementary Table 2 . Since endoderm formation was not enriched in the GO biological process categories for HEB/PRC2, we compared our gene lists to a hand-curated list of 51 definitive endoderm (DE) genes [36] , [37] . Of the 51 DE genes, 41 are bound by HEB/PRC2, but only four are bound by PRC2 alone and six are not bound by either factor ( Fig. 1g and Supplementary Fig. 1e ). The list of genes containing HEB/PRC2 promoters includes known mesoderm and endoderm (ME) regulators such as Sox17 , Gata4 , Gata6 , Wnt3a , Foxa2 , Brachyury ( T ), Pitx2 , Eomes , Gsc and Hand1 , and HEB binding to these genomic loci is clearly shown to be associated with PRC2 components such as SUZ12, EZH2 and JARID2 ( Supplementary Fig. 1f ). In contrast, the Lefty2 promoter is not associated with PRC2 but is bound by both HEB and SMAD2/3, suggesting that it is not repressed. Furthermore, HEB/PRC2 promoters mark members of the Hox (38) and Fox (19) gene families, which are not found in the gene set marked by PRC2 alone ( Fig. 1g ). Overall, our data suggest that HEB associates with a distinct subset of PRC2-bound promoters that specifically function to drive mesoderm and endoderm fates, and importantly mark the promoters of both Hox and Fox family members. HEB is necessary for SMAD2/3 chromatin association We functionally examined the role of HEB in mouse ESCs. To this end, we depleted HEB in ESCs using lentivirus-mediated shRNA which specifically depleted HEB transcripts resulting in a significant reduction of protein (<5% remain) ( Fig. 2a and Supplementary Fig. 2a ) in both the nucleus and cytoplasm compared with control shRNA infected cells ( Supplementary Fig. 2b ). The expression of the pluripotency genes, Oct4 and Nanog , and OCT4 protein levels in the nucleus was similar in HEB-depleted ESCs compared with controls. However, we do observe an increase in LEFTY in the cytoplasm of HEB-depleted ESCs ( Fig. 2a and Supplementary Fig. 2b ). Also, the morphology of HEB-depleted ESCs was no different from controls and the cells maintained an undifferentiated appearance through multiple passages (five passages; Supplementary Fig. 2c ). Figure 2: Depletion of HEB drives ME differentiation. ( a ) Western blot analysis on control shRNA (shCont) and shHEB-treated mouse ESCs detected the protein expression of HEB, LEFTY and OCT4. TUBULIN was used for loading control. ( b – f ) Chromatin immunoprecipitation (ChIP) using anti-HEB ( b ), E2A ( c ), SMAD2/3 ( d ), H3K27me3 ( e ) and JARID2 ( f ) antibodies in either shCont (green) or shHEB (orange) ESCs. Pulled-down chromatin was analysed by qPCR using primers surrounding distal enhancer regions of Lefty1 , Lefty2 and Id1 and proximal promoter regions of Brachyury ( T ) and Sox9 , which are occupied by PRC2 in mouse ESCs. The Actb locus was used as a negative control. Error bars are based on the s.d. derived from triplicate qPCR reactions and enrichment is calculated relative to input. * P <0.05 by Student’s paired t -test with a two-tailed distribution. ( g ) Western analysis of HEB, GATA4, SOX17, LEFTY and SMAD2/3 in EBs after 4 days of differentiation from shCont or shHEB ESCs at different concentrations of Activin (0–100 ng ml −1 ) treatment. TUBULIN was used as a loading control. ( h ) qPCR with reverse transcription analysis of 4-day EBs derived from shCont (blue) or shHEB (pink) ESCs either without Activin (0 ng ml −1 ) or a low dose of Activin (5 ng ml −1 ). Expression was normalized to Gapdh transcript levels. Error bars represent s.d. calculated from triplicate qPCR reactions. Full size image To validate the anti-HEB antibody that we used for ChIP analysis, ESCs targeted with shCont or shHEB were immunoprecipitated with rabbit anti-HEB antibody and probed with mouse anti-HEB antibody, which incidentally did not work for ChIP in our hands. Precipitated HEB was detected, as a single band, by pull down using both the anti-HEB and anti-E2A antibodies in controls, but not in shHEB cells. As HEB and E2A form heterodimers, it is not surprising that HEB was detected when precipitating using anti-E2A ( Supplementary Fig. 2d ). To determine whether HEB is still bound to chromatin in knockdown cells, we examined HEB-depleted (shHEB) and control (shCont) ESCs using ChIP-qPCR (quantitative PCR) for HEB occupancy at genomic regions displaying different protein combinations: Distal enhancer regions of Lefty1 and Lefty2 are bound by both SMAD2/3 and HEB, a distal region of Id1 is only bound by HEB, and promoter regions of Brachyury ( T ) and Sox9 are bound by PRC2 and HEB. In shHEB cells, we found that HEB binding was significantly decreased at the distal elements near Lefty1 , Lefty2 and Id1 compared with controls ( Fig. 2b ). SMAD2/3, as well as E2A, binding was also significantly reduced at the Lefty1 and Lefty2 distal loci, suggesting that SMAD2/3 and E2A are dependent on HEB for chromatin association ( Fig. 2c,d ). Conversely, HEB was not significantly depleted at the PRC2-bound promoter regions of Brachyury ( T ) and Sox9 . We also observed no effect on H3K27me3 and JARID2 levels at the Brachyury ( T ) and Sox9 promoters ( Fig. 2e,f ). This suggests that HEB binding at chromatin is stronger when associated with PRC2 components than at distal elements. Importantly, this also demonstrates that HEB depletion in mouse ESCs results in a hypomorphic phenotype, which may be masking a more severe effect. HEB knockdown induces premature ME gene transcription To further examine the developmental potential of HEB-depleted mouse ESCs, we differentiated shHEB and shCont cells into embryoid bodies (EBs) over a 4-day period ( Supplementary Fig. 3 ), an in vitro assay that mimics the early stages of germ layer development. On day 2 of the assay, we added different concentrations of Activin (0, 5, 25 and 100 ng ml -1 ) which is known to drive cells toward the mesoderm and endoderm lineages On day 4, we examined GATA4, SOX17 and LEFTY protein levels, known markers for mesodermal and endodermal differentiation, using western blotting. We found that GATA4 and SOX17 were induced in HEB-depleted EBs even in the absence of Activin (0 ng ml -1 , Fig. 2g ). At all concentrations of Activin, GATA4 is more highly expressed in the shHEB-treated EBs compared with controls. LEFTY protein was not preferentially induced in shHEB differentiated EBs, except at the highest dose of Activin. This appears contradictory to what we observe in ESCs as LEFTY is highly expressed when HEB is depleted. It is likely that HEB, while being a critical repressor of Lefty in ESCs, no longer has that role in differentiated cells where Lefty is only responsive to high doses of Activin. In parallel, we examined EBs exposed to either 5 ng ml -1 or no Activin using qPCR with reverse transcription for Gata4 , Brachyury ( T ) and Foxa2 ( Fig. 2h ). We found strong induction of Brachyury ( T ) , Foxa2 and Gata4 in shHEB EBs in the absence of Activin compared with controls. Of note, Heb mRNA reduction was well validated in the shHEB-treated cells, while Smad2 and Actb mRNA levels were unchanged. To characterize global transcription profiles after HEB knockdown, we performed 3SEQ with biological triplicates of shHEB and shControl in three different cell types: ESCs, EBs without Activin (0 ng ml -1 ) and EBs with Activin (100 ng ml -1 ) ( Supplementary Fig. 4 ). In each cell type, we identified transcripts whose abundance differed at least twofold between shHEB and shControl, with a significance threshold of Benjamini–Hochberg-corrected P <0.1. The transcripts that meet these criteria, either upregulated or downregulated, are listed in Supplementary Data 1 . In ESCs depleted for HEB, we see little evidence of transcriptional change. In shHEB ESCs, 37 transcripts were downregulated and 42 transcripts were upregulated compared with shControl ( Supplementary Fig. 4a ). Although the LEFTY protein is increased in shHEB ESCs, the transcript level was not significant in the biological triplicate (1.4-fold increase, P >0.2), suggesting that there may be an additional posttranscriptional regulation occurring. We found little functional significance in any of these ESCs groups although the downregulated transcripts were enriched for ‘cellular amino acid and derivative metabolic process’ (DAVID GO:0006519, P >0.003). Overall, HEB-depleted ESCs have few changes from control ESCs, although it is important to consider that HEB is still bound to promoters in ESCs and therefore may still be functional. Unlike the ESCs scenario, we found significant changes between shHEB and shControl transcripts in EBs differentiated in the absence of Activin ( Supplementary Fig. 4b ): 531 transcripts were downregulated and 561 upregulated in HEB knockdown cells. Using DAVID GO, we find significant enrichment for ‘developmental process’ (up, P =4.50E-29; down, P =2.30E-08; Supplementary Fig. 4d ). Brachyury ( T ), Eomes , Gata4 , Gsc , Foxa2 and Sox17 were among the transcripts increased in the shHEB EBs without Activin, suggesting that HEB knockdown induced expression of many mesoderm- and endoderm-related genes in the absence of Nodal or Activin signals. Confirming this observation, shHEB EBs treated with high doses of Activin showed 706 downregulated transcripts and 831 upregulated transcripts. These upregulated transcripts include Eomes , Gata4 , Gata6 , Gsc and Sox17 and are significant for the term ‘developmental process’ (up, P =4.61E-16; Supplementary Fig. 4e ). Overall, our data shows that HEB depletion leads to mesoderm and endoderm induction in the absence of Activin or Nodal signals. HEB/SMAD2/3 elements correspond with enhancer marks As we found that HEB binds PRC2 at developmental promoters, we next examined how this binding might correlate with Nodal signalling. To this end, we examined the overlap between SMAD2/3- and HEB-bound regions and found that 83% of the SMAD2/3-bound regions (3,414/4,111) are also bound by HEB ( Fig. 3a , Supplementary Fig. 5a and Supplementary Table 1 ). Further, when we examined the role of genes that neighbour HEB/SMAD2/3 elements using GREAT, a programme that predicts the function of cis-regulatory elements [34] , we found a significant enrichment for developmental processes (Binom raw, P =1.72E-138; Supplementary Fig. 5b ). To determine the extent of overlap between HEB/SMAD2/3 elements and HEB/PRC2 promoters in ESCs, we compared regions occupied by SMAD2/3, SUZ12 or HEB. While we found that many HEB-bound sites are co-occupied by SMAD2/3 (see above), <2% (77/4,111) of SMAD2/3-bound loci are also bound by SUZ12 ( Fig. 3a ; similar observation is found with EZH2, data not shown). This observation is consistent with our co-immunoprecipitation data showing that SMAD2/3 does not interact with JARID2, EZH2 or H3K27me3 in ESCs ( Fig. 1d ). Furthermore, when we examine the genomic distribution of the 3,324 regions bound by both SUZ12 and EZH2 ( Fig. 1c ) and the 3,414 regions bound by both HEB and SMAD2/3, we find that SUZ12/EZH2 most frequently binds within a 5 kb of the TSS, whereas HEB/SMAD2/3 binds 5–50 kb from the TSS ( Fig. 3b ). 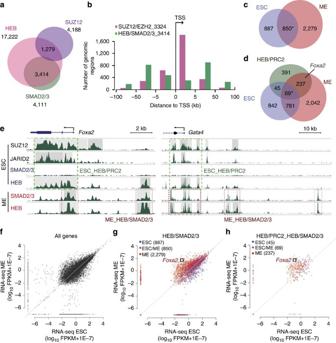Figure 3: HEB/PRC2 in ESCs are replaced by HEB/SMAD2/3 in ME. (a) Venn diagram comparing the overlap between HEB, SUZ12 and SMAD2/3 binding genome wide with a threshold >1 bp overlap between bound peak regions. (b) Histogram showing the number of genomic regions bound by both SUZ12 and EZH2 (pink; 3,324) and regions bound by both HEB and SMAD2/3 (green; 3,414) with respect to the distance from a neighbouring TSS at 0–5, 5–50 and 50–100 kilobase (kb) intervals. (c) Venn diagram demonstrating the overlap of genes that neighbour both HEB and SMAD2/3-bound regions within 50 kb from a TSS in ESC (1,737 (887+850) genes; blue) and ME (3,129 (2,279+850) genes; orange) (*P<1.0E-325). Significance was tested using Fisher’s exact test. (d) The overlap of genes containing HEB/PRC2 promoters in ESC (742 (391+237+69+45) genes; green) with the genes associated to HEB/SMAD2/3 elements in either ESC (1,737 (842+781+69+45) genes; blue) or ME (3,129 (2,042+781+69+237) genes; orange) (*P<1.0E-14).Foxa2is highlighted as an example of a gene with overlapping HEB/PRC2 promoters and HEB/SMAD2/3 elements only in ME. (e) Genome browser representation of theFoxa2andGata4genomic loci as examples of genes overlapping HEB/PRC2 promoters and HEB/SMAD2/3 elements in ME. Only HEB is co-bound with SUZ12 and JARID2 near to the TSS in ESCs (ESC_HEB/PRC2; green dotted box), but in ME, newly made HEB/SMAD2/3 elements are shown near to the TSS as well as a distal region (ME_HEB/SMAD2/3; red dotted boxes). (f–h) Scatterplots comparing RNA-seq expression data between mouse ESCs (ESC) and Activin-treated differentiated ME. Each dot corresponds to one NCBI Reference Sequence (RefSeq) transcript with expression measured as fragments per kilobase of transcript per million mapped reads (FPKM). (f) All genes aligned from RNA-seq data in both cell types. The grey line in each scatterplot represents no difference in gene expression between cell types. (g) Expression comparison of genes that neighbour HEB/SMAD2/3 elements within 50 kb from a TSS only in ESCs (ESC, 887 genes), in both ESC and ME (ESC/ME, 850 genes) and only ME (ME, 2,279 genes). (h) Expression comparison of genes containing both HEB/PRC2 promoters and HEB/SMAD2/3 elements only in ESC (ESC, 45 genes), both in ESC and ME (ESC/ME, 69 genes) and only in ME (ME, 237 genes). Figure 3: HEB/PRC2 in ESCs are replaced by HEB/SMAD2/3 in ME. ( a ) Venn diagram comparing the overlap between HEB, SUZ12 and SMAD2/3 binding genome wide with a threshold >1 bp overlap between bound peak regions. ( b ) Histogram showing the number of genomic regions bound by both SUZ12 and EZH2 (pink; 3,324) and regions bound by both HEB and SMAD2/3 (green; 3,414) with respect to the distance from a neighbouring TSS at 0–5, 5–50 and 50–100 kilobase (kb) intervals. ( c ) Venn diagram demonstrating the overlap of genes that neighbour both HEB and SMAD2/3-bound regions within 50 kb from a TSS in ESC (1,737 (887+850) genes; blue) and ME (3,129 (2,279+850) genes; orange) (* P <1.0E-325). Significance was tested using Fisher’s exact test. ( d ) The overlap of genes containing HEB/PRC2 promoters in ESC (742 (391+237+69+45) genes; green) with the genes associated to HEB/SMAD2/3 elements in either ESC (1,737 (842+781+69+45) genes; blue) or ME (3,129 (2,042+781+69+237) genes; orange) (* P <1.0E-14). Foxa2 is highlighted as an example of a gene with overlapping HEB/PRC2 promoters and HEB/SMAD2/3 elements only in ME. ( e ) Genome browser representation of the Foxa2 and Gata4 genomic loci as examples of genes overlapping HEB/PRC2 promoters and HEB/SMAD2/3 elements in ME. Only HEB is co-bound with SUZ12 and JARID2 near to the TSS in ESCs (ESC_HEB/PRC2; green dotted box), but in ME, newly made HEB/SMAD2/3 elements are shown near to the TSS as well as a distal region (ME_HEB/SMAD2/3; red dotted boxes). ( f – h ) Scatterplots comparing RNA-seq expression data between mouse ESCs (ESC) and Activin-treated differentiated ME. Each dot corresponds to one NCBI Reference Sequence (RefSeq) transcript with expression measured as fragments per kilobase of transcript per million mapped reads (FPKM). ( f ) All genes aligned from RNA-seq data in both cell types. The grey line in each scatterplot represents no difference in gene expression between cell types. ( g ) Expression comparison of genes that neighbour HEB/SMAD2/3 elements within 50 kb from a TSS only in ESCs (ESC, 887 genes), in both ESC and ME (ESC/ME, 850 genes) and only ME (ME, 2,279 genes). ( h ) Expression comparison of genes containing both HEB/PRC2 promoters and HEB/SMAD2/3 elements only in ESC (ESC, 45 genes), both in ESC and ME (ESC/ME, 69 genes) and only in ME (ME, 237 genes). Full size image To determine whether HEB/SMAD2/3 elements also contained chromatin-enhancer marks, we examined previously published ChIP-seq data in ESCs for H3K27ac, H3K4me1 and p300 (ref. 38 ). Among the 3414 HEB/SMAD2/3 elements, 2015 regions overlapped with high-occupancy sites of H3K27ac, 1002 regions with H3K4me1 and 2902 regions with p300 ( Supplementary Fig. 5c–e ). If we then overlap HEB/SMAD2/3, p300 and H3K27ac, we find 1821 regions associated with all four components. Further, if we ask for regions containing HEB/SMAD2/3, p300, H3K27ac and H3K4me1, we find 671. The extent of this overlap is illustrated at the Lefty1 locus ( Supplementary Fig. 5f ). Overall, this strongly validates that many of the HEB/SMAD2/3-occupied regions are in the correct chromatin conformation to be considered as likely enhancer elements. To further validate that the HEB/SMAD2/3-occupied regions may function as enhancers, we found three well-characterized Activin response elements (AREs) in the literature, including Pitx2 , Otx2 and Lefty2 (refs 39 , 40 , 41 ). When we compare these regions to the HEB/SMAD2/3 elements—all three directly overlap in ME ( Supplementary Fig. 6 ). Interestingly, Pitx2 is one of the 53 genes ( Supplementary Table 3 ) that has HEB/PRC2 promoter in ESCs and HEB/SMAD2/3 element in ME and the mouse ARE precisely overlaps with this HEB/SMAD2/3 element. Further, all three of these AREs also can be found in X . tropicalis where they are associated with H3K4me1 and H3K27ac chromatin-enhancer marks, suggesting evolutionarily conserved function [42] . Overall, this strongly suggests that the HEB/SMAD2/3 enhancers are indeed functional. HEB/SMAD2/3 elements are linked with HEB/PRC2 We next asked whether HEB and SMAD2/3 occupancy changes during differentiation. To address this question, we used ChIP-seq with anti-HEB and anti-SMAD2/3 antibodies on EBs that were treated with a high dose of Activin (100 ng ml -1 ; Supplementary Fig. 3 ; referred to as mesoderm and endoderm or ME). We found that a majority (61%; 6,703/11,033) of SMAD2/3-bound regions were also bound by HEB ( Supplementary Table 1 and Supplementary Fig. 5g ), an observation that we also noted in our analysis of ESCs. Intriguingly, only 14% (944/6,703) of these sites were shared between the two data sets (ESC versus ME), suggesting that 5,759 new loci are bound by HEB and SMAD2/3 during ME differentiation ( Supplementary Fig. 5h ). Additional analysis indicates that HEB/SMAD2/3-bound elements in ME are associated with 3,129 genes (defined as nearest neighbouring gene within 50 kb of the TSS), of which only 850 are also associated with HEB/SMAD2/3 binding in ESCs ( Fig. 3c ). These genes are listed in Supplementary Data 2 . Next, we examined the transcriptional levels of genes associated with HEB/SMAD2/3 elements using previously published RNA-seq data ( Fig. 3f,g ) [43] . We found that the 3,129 genes associated with HEB/SMAD2/3 elements in ME had a significantly greater average increase in expression level than the 887 genes associated with HEB/SMAD2/3 elements in ESC using Welch’s one-sided two-sample t -test ( P <2.20E-16; Fig. 3g and Supplementary Fig. 7a ), suggesting that the newly formed enhancers are more active. As HEB/SMAD2/3 elements and HEB/PRC2-bound promoters are both highly enriched at developmental genes, we next tested whether these enhancers and promoters might target the same genes. To this end, we compared genes containing HEB/PRC2 promoters in ESC (742) with those associated to HEB/SMAD2/3 elements in either ESC (1,737 genes) or in ME (3,129 genes) at a distance of 50 kb from TSS ( Fig. 3d ; see similar analysis for 2 kb distance in Supplementary Fig. 5i ). We found that 41% (306/742) of the genes with HEB/PRC2-marked promoters become associated with HEB/SMAD2/3 elements in ME, while only 15% (114/742) of the HEB/PRC2-marked genes are associated with similar elements in ESC ( Fig. 3d ). For example, both Foxa2 and Gata4 have a HEB/PRC2-bound promoter in ESC, which are subsequently associated with a HEB/SMAD2/3 element in ME ( Fig. 3e ). This is suggestive that HEB may serve to connect the SMAD2/3 signalling to the promoter upon differentiation. If HEB does serve as a link between these developmental promoters and Nodal target enhancers, then it should confer function at these loci. To this end, we compared the transcript levels of 45 genes in ESC, 69 in both ESC and ME and 237 genes in ME, all of which had promoters occupied by HEB/PRC2 in ESC that subsequently became associated with a HEB/SMAD2/3. We found that the genes associated with HEB and SMAD2/3 binding during ME differentiation had a significantly greater average increase in expression levels than those associated only in ESC using Welch’s one-sided two-sample t -test ( P =9.14E-8; compare Fig. 3g with 3 h and Supplementary Fig. 7a,b ). To elucidate whether this difference is due to the presence of SMAD2/3, but not HEB, we performed the same analysis but compared the expression of genes associated with PRC2 in ESCs and SMAD2/3 element without HEB ( Supplementary Data 3 ). Given these parameters, we find 16 genes only in ESCs, 23 genes in both ESCs and ME and 357 genes only in ME. We find significant expression differences in genes that contain PRC2-occupied promoters in ESCs and SMAD2/3-bound elements in ME ( P =8.27E-8). However, in the absence of HEB, we find that expression does not change between ESC and ME ( P =0.5351, Supplementary Fig. 7c,d ). Overall, this strongly suggests that HEB is a major driver of transcriptional activity and that SMAD2/3 is not as effective as HEB/SMAD2/3 in effecting downstream transcriptional responses. HEB/SMAD2/3 replaces HEB/PRC2 regions at ME loci We have shown that HEB/PRC2-marked promoters become associated with HEB/SMAD2/3 elements after differentiation into ME and that the presence of HEB is essential for transcriptional activity at these loci. We next asked whether HEB/PRC2 promoters in ESCs are actually replaced by HEB/SMAD2/3 binding during ME differentiation. We identified 53 genes that have promoters bound by HEB/PRC2 in ESCs as well as HEB/SMAD2/3 in ME. This is illustrated at the Foxa2 and Gata4 loci where a broad domain of SUZ12, JARID2 and HEB exists at the promoter in ESC, and is replaced by HEB/SMAD2/3 binding upon ME differentiation ( Fig. 3e ). Additional genes that undergo this replacement include Gata6, Gsc, Fgf5 , Lhx1 and Pitx2 ( Supplementary Table 3 for complete list). This suggests that HEB/SMAD2/3 replaces HEB/PRC2 at a subset of promoters upon differentiation at key mesodermal and endodermal loci. While we only observe 53 of these promoters, we suggest that many more would exist within the differentiation regime and that we are simply capturing those present at the time period we examined. EED is required for HEB deposition We next tested whether PRC2 is required for HEB binding at developmental promoters. To this end, we examined HEB occupancy in Eed homozygous mutant ( Eed -/-) ESCs, which have disruption of PRC2-mediated H3K27 methylation, but can maintain ESC pluripotency on mouse embryonic fibroblasts (MEFs) [7] , [25] , [26] , [35] , [44] ( Supplementary Fig. 8a,b ). Using western blot analysis and ChIP-qPCR, we show that Eed -/- ESCs lack EED protein in total lysates or bound to chromatin ( Fig. 4a and Supplementary Fig. 8c,d ) have reduced protein levels of H3K27me3 and EZH2, but maintain SUZ12 and JARID2, consistent with previous reports [7] , [35] . We note that the levels of HEB and other components of the Nodal signalling pathway (including SMAD2/3 and LEFTY) were unchanged in Eed -/- cells compared with wild-type control. 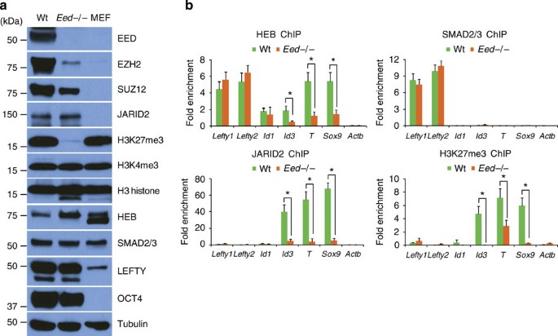Figure 4: HEB binding to developmental promoters is dependent on PRC2. (a) Western blot analysis from wild-type E14 ESCs (Wt),Eed-/- mutant cells (Eed-/-) or MEF lysates depicting the presence of EED, EZH2, SUZ12, JARID2, H3K27me3, H3K4me3, total H3 histone, HEB, SMAD2/3, LEFTY and OCT4. TUBULIN was used for loading control. (b) ChIP-qPCR to determine whether HEB, SMAD2/3, JARID2 and H3K27me3 associate with chromatin in the absence of EED. ChIP was performed using anti-HEB, SMAD2/3, JARID2 and H3K27me3 antibodies from wild-type E14 (green) orEed-/- (orange) ESCs. The pulled-down chromatin was then analysed by qPCR using primers surrounding the distal SMAD2/3-boundLefty1andLefty2regions and the promoter PRC2-bound elements at theBrachyury(T) andSox9promoters. BothId1andId3are used for positive control for HEB binding, but onlyId3is used for positive target of both PRC2 and H3K27me3. Error bars represent s.d. calculated from triplicate qPCR reactions. Fold enrichment was calculated relative to input andActblocus was served as a negative control. *P<0.05 by Student’s pairedt-test with a two-tailed distribution. Figure 4: HEB binding to developmental promoters is dependent on PRC2. ( a ) Western blot analysis from wild-type E14 ESCs (Wt), Eed -/- mutant cells ( Eed -/-) or MEF lysates depicting the presence of EED, EZH2, SUZ12, JARID2, H3K27me3, H3K4me3, total H3 histone, HEB, SMAD2/3, LEFTY and OCT4. TUBULIN was used for loading control. ( b ) ChIP-qPCR to determine whether HEB, SMAD2/3, JARID2 and H3K27me3 associate with chromatin in the absence of EED. ChIP was performed using anti-HEB, SMAD2/3, JARID2 and H3K27me3 antibodies from wild-type E14 (green) or Eed -/- (orange) ESCs. The pulled-down chromatin was then analysed by qPCR using primers surrounding the distal SMAD2/3-bound Lefty1 and Lefty2 regions and the promoter PRC2-bound elements at the Brachyury ( T ) and Sox9 promoters. Both Id1 and Id3 are used for positive control for HEB binding, but only Id3 is used for positive target of both PRC2 and H3K27me3. Error bars represent s.d. calculated from triplicate qPCR reactions. Fold enrichment was calculated relative to input and Actb locus was served as a negative control. * P <0.05 by Student’s paired t -test with a two-tailed distribution. Full size image To determine whether HEB occupancy at both promoters and distal elements is dependent on PRC2, we performed ChIP using anti-HEB, anti-SMAD2/3, anti-JARID2 and anti-H3K27me3 antibodies on wild-type or Eed -/- ESCs followed by qPCR for the Lefty1 , Lefty2 , Id1 , Id3 , Brachyury ( T ) and Sox9 loci. Interestingly, at loci such as Lefty1 and Lefty2 in which both HEB and SMAD2/3 bind to distal enhancer elements, HEB binding is unaffected in EED mutants. However, at the Brachyury ( T ) and Sox9 promoters, which are bound by the HEB/PRC2, HEB occupancy is dependent on EED ( Fig. 4b ). Similarly, JARID2 and H3K27me3 occupancy are highly dependent upon the presence of EED at Brachyury ( T ) and Sox9. Overall, we suggest that HEB is dependent on EED for occupancy at promoters, but not at HEB/SMAD2/3 elements in ESCs. HEB dependency on Nodal is cell specific We next examined whether HEB occupancy is dependent on Nodal signalling in mouse ESCs. Therefore, we treated ESCs for 24 or 48 h with SB431542, a drug that inhibits the phosphorylation of SMAD2/3 (ref. 45 ). After SB431542 treatment, ESCs exhibit normal morphology ( Fig. 5a ), which is consistent with previous work showing that Nodal signalling is not necessary for mouse ESC pluripotency [46] , [47] . However, SB431542 treatment results in a significant decrease in phosphorylated SMAD2 (pSMAD2) and LEFTY ( Fig. 5b ), suggesting that Nodal signalling is indeed compromised. 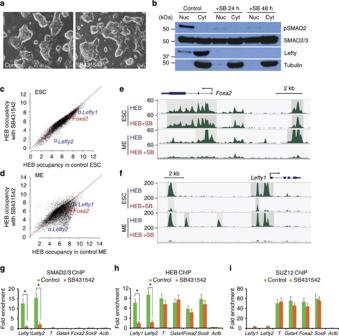Figure 5: HEB/PRC2 is Nodal independent, but HEB/SMAD2/3 is Nodal dependent. (a) Morphology of control (left) and SB431542-treated (right) mouse ESCs. (b) Nodal signalling is compromised after 24-h treatment with SB431542 (SB). Western blot showing phosphorylated SMAD2 (pSMAD2), total SMAD2/3 and LEFTY protein expression in the nuclear (Nuc) and cytoplasmic (Cyt) fraction of ESCs treated without (control) or with SB431542 (SB) for 2 or 48 h. TUBULIN was used for loading control and as a cytoplasmic-specific marker. (c,d) Scatterplots of ChIP-seq data showing HEB occupancy without (control) or with SB431542 treatment in ESC (c) and ME (d). The red line in each scatterplot represents no change in HEB binding on SB431542 treatment in each cell type.Lefty1,Lefty2andFoxa2loci are boxed. (e,f) The genome browser representations of HEB binding toFoxa2(e) andLefty1(f) genomic loci upon SB431542 treatment are shown for ESC and ME. (g–i) ChIP-qPCR using anti-SMAD2/3 (g), anti-HEB (h) and anti-SUZ12 (i) antibodies to pull down chromatin in either control (green) or SB431542-treated (orange) ESCs. Occupancy of these factors was then determined at theLefty1,Lefty2,Brachyury(T),Gata4,Foxa2andSox9regions. TheActblocus served as a negative control. Error bars represent s.d. calculated from triplicate qPCR reactions. Fold enrichment was calculated relative to input. *P<0.05 by Student’s pairedt-test with a two-tailed distribution. Figure 5: HEB/PRC2 is Nodal independent, but HEB/SMAD2/3 is Nodal dependent. ( a ) Morphology of control (left) and SB431542-treated (right) mouse ESCs. ( b ) Nodal signalling is compromised after 24-h treatment with SB431542 (SB). Western blot showing phosphorylated SMAD2 (pSMAD2), total SMAD2/3 and LEFTY protein expression in the nuclear (Nuc) and cytoplasmic (Cyt) fraction of ESCs treated without (control) or with SB431542 (SB) for 2 or 48 h. TUBULIN was used for loading control and as a cytoplasmic-specific marker. ( c , d ) Scatterplots of ChIP-seq data showing HEB occupancy without (control) or with SB431542 treatment in ESC ( c ) and ME ( d ). The red line in each scatterplot represents no change in HEB binding on SB431542 treatment in each cell type. Lefty1 , Lefty2 and Foxa2 loci are boxed. ( e , f ) The genome browser representations of HEB binding to Foxa2 ( e ) and Lefty1 ( f ) genomic loci upon SB431542 treatment are shown for ESC and ME. ( g – i ) ChIP-qPCR using anti-SMAD2/3 ( g ), anti-HEB ( h ) and anti-SUZ12 ( i ) antibodies to pull down chromatin in either control (green) or SB431542-treated (orange) ESCs. Occupancy of these factors was then determined at the Lefty1 , Lefty2 , Brachyury ( T ), Gata4 , Foxa2 and Sox9 regions. The Actb locus served as a negative control. Error bars represent s.d. calculated from triplicate qPCR reactions. Fold enrichment was calculated relative to input. * P <0.05 by Student’s paired t -test with a two-tailed distribution. Full size image We next perfosrmed ChIP-seq using anti-HEB antibodies on SB431542-treated ESCs and ME (for sequencing numbers see Supplementary Table 1 ). Using UniPeak [48] , we compared HEB occupancy across the genome in control and SB431542-treated ESCs and ME ( Fig. 5c,d ). Interestingly, HEB occupancy was unaffected by Nodal inhibition at most loci in ESC ( r =0.96), including at the Foxa2 locus ( Fig. 5c , red box; Fig. 5e , ESC genome browser shot). There are, however, a few notable loci, such as Lefty1 and Lefty2 that are Nodal dependent ( Fig. 5c , blue boxes; Fig. 5f , ESC genome browser shot). To validate our results, we performed ChIP-qPCR using anti-SMAD2/3, anti-HEB and anti-SUZ12 on control and SB431542-treated ESCs ( Fig. 5g–i ). We then amplified HEB-bound loci that we found to be Nodal dependent ( Lefty1 and Lefty2 ) or Nodal independent ( Brachyury ( T ), Gata4 , Foxa2 and Sox9— all of which contain HEB/PRC2 promoters). Our ChIP-qPCR analysis confirms that SMAD2/3 and HEB occupancy at the Lefty1 and Lefty2 regions are indeed Nodal dependent, yet at most loci, HEB/PRC2 deposition is independent of Nodal signalling in ESCs. To examine whether HEB occupancy was dependent upon Nodal signalling in differentiated ME, we compared HEB occupancy in Activin-treated EBs (ME) with or without SB431542 using ChIP-seq with an anti-HEB antibody. Unlike HEB occupancy in mouse ESCs, Nodal inhibition caused widespread HEB depletion in SB431542-treated day 4 EBs ( r =0.65) at both promoters and SMAD2/3-bound elements ( Fig. 5d ). Genome browser shots of the Foxa2 and Lefty1 loci demonstrate that HEB-bound elements, including both distal elements and promoters, in ME are highly dependent on Nodal signals ( Fig. 5e,f ). Overall, our data confirm that, in differentiated ME, HEB binding is globally dependent on Nodal signalling, while, in ESCs, HEB is dependent on Nodal signalling only in the context of a few HEB/SMAD2/3 elements and its role as a PRC2 component is distinct and independent of Nodal. Here we demonstrate that HEB links the PRC2-mediated repression of mesodermal and endodermal specific promoters to their subsequent activation by the Nodal signalling pathway. Our data suggest that HEB together with PRC2 enables the selective targeting of these critical promoters by Nodal signalling. In support of this, we find that most of the known mesoderm and endoderm regulatory pathway members contain HEB/PRC2-bound promoters in mouse ESCs which become associated with a HEB/SMAD2/3 element upon differentiation. Intriguingly, we also find that many HEB/PRC2-bound promoters, including those of the genes Gata4, Gata6, Gsc, Foxa1, Foxa2, Foxq1 , Bmp7 , Fgf5 , Fgfr2 , Lhx1 , Lef1 , Pitx2 and 41 others, become occupied by HEB/SMAD2/3 after Activin exposure, suggesting that HEB may function as a dock for enhancers. All of these loci have the same hallmarks of activation but we will use Gata4 to illustrate the observed scenario: the Gata4 promoter is occupied by the HEB/PRC2 complex in ESCs, but when we deplete HEB from ESCs and then differentiate into EBs, Gata4 becomes expressed even without Activin—demonstrating that the promoter has been activated ( Supplementary Fig. 9a ). In addition, when we examine HEB occupancy in ME, we find that the Gata4 promoter has maintained HEB occupancy, lost the PRC2 complex and gained SMAD2/3. Further, HEB and SMAD2/3 co-localize at a newly formed putative enhancer element around 10 kb from the Gata4 promoter region. The proximity of a HEB/SMAD2/3 promoter and HEB/SMAD2/3 regulatory element implies that these regions may interact and provides a potential mechanism for activation of these important lineage-specific genes ( Supplementary Fig. 9b ). In support of a model where HEB cooperates with PRC2 to effectively mark developmental promoters for eventual SMAD2/3 occupancy, SMAD2/3 has been shown to recruit the demethylase JMJD3 to the Nodal promoter, suggesting a mechanism for alleviating H3K27me3 repression at this locus [31] . We suggest that when poised promoters are exposed to high levels of extrinsic Nodal signals, JMJD3 might be central to the derepression of the HEB/PRC2 complex with HEB serving as a dock for SMAD2/3 at these selective developmental promoters. Overall, it will be interesting to investigate whether the presence of HEB serves to allow SMAD2/3/JMJD3 to target PRC2 promoters. If HEB enables SMAD2/3/JMJD3 to specifically target developmental promoters on the first extrinsic differentiation cue, then a similar mechanism, but with different mediators, might exist for other lineages. PRC2 could cooperate with different proteins that allow signalling pathways to interface with ectodermal or trophectodermal promoters. To investigate this, we have examined the ENCODE and GEO data sets for localization of other HLH proteins, including MYOD and ASCL1, but we have not observed any that overlap with PRC2 genome-wide. However, as these data sets are currently limited, this requires further investigation. Regardless, we propose that HEB is necessary to restrict differentiation of mesoderm and endoderm from mouse ESCs and does so in conjunction with PRC2. While we find an important role for HEB in repressing initial differentiation events from a stem cell population, mouse mutations in this locus are viable. In the mouse, the roles of HEB and its family members E2A and E2-2, have been extensively characterized as essential factors in hematopoiesis. The phenotypes of single-gene knockout models for E2A and HEB demonstrated that E2A was the primary E-protein member driving B-cell development, but that both E2A and HEB were required for proper T-cell development [49] , [50] , [51] , [52] . As the HEB homozygous null mice die after birth, it seems contradictory that HEB might have a role in the transition from pluripotency to germ layer formation. However, mouse ESCs are an in vitro model system that is most certainly not precisely similar to any state that exists in the mouse embryo. There are several examples of molecules being essential for pluripotency and early differentiation in mouse ESCs, but yet the genetic mouse mutant has no deficits during cognate in vivo stages. Esrrb has been shown to be a necessary target of both NANOG and GSK3 and is known to mediate the maintenance of pluripotency in mouse ESCs [53] , [54] . However, mouse mutants for Esrrb die at midgestation due to chorionic and placental defects, not due to embryonic failure [55] . Like ESRRB, LIF is critical in maintaining mouse ESCs, but the mouse mutation survives embryogenesis with impairments in stem cell populations of the immune system, not unlike HEB [56] . In addition, the fact that HEB functions as a heterodimer with a multitude of HLH proteins suggests that the precise cellular context matters [57] , [58] . One could imagine that in ESCs, HEB has adopted the ability to form homodimers at promoters, but within the embryo, another HLH might act together with HEB to elicit this same function. As there is clearly genetic redundancy between these E proteins, particularly E2A, HEB and E2-2, compound mutations are needed to study the role of this family during embryogenesis. We hypothesize that HEB occupancy at the PRC2 promoters serves as an important dock for eventual SMAD2/3 promoter association. Whether HEB directly serves in a repressive context at the PRC2 promoters in mouse ESCs is still an open question as HEB depletion did not lead to a reduction in HEB or PRC2 components at these locations, therefore, we cannot accurately assess its role. However, on exposure to extrinsic signals to drive differentiation, HEB is required for the repression of mesendodermal promoters, suggesting that it may indeed serve this role in mouse ESCs. Interestingly, in mouse ESCs, HEB associates with PRC2 at mesodermal, endodermal, Hox and Fox promoters in a Nodal-independent fashion, suggesting that chromatin is marked before Nodal exposure. Conversely, HEB occupancy at these regions depends on PRC2 as HEB cannot associate to developmental promoters in the absence of EED. This suggests that while Nodal is dispensable for HEB association to developmental promoters, PRC2 is essential and adds support for the idea that HEB may indeed function as part of this complex. Overall, the presence of HEB at both PRC2-bound promoters and SMAD2/3-bound enhancers and the functional role of HEB in mesodermal and endodermal lineages strongly suggests that there is an interplay between these components with HEB performing repressive or activating roles depending upon the cellular context and the concentration of Nodal signals. Future investigation will be required to elucidate the mechanisms by which HEB controls the poised nature of both enhancers and promoters. Cell culture Mouse CGR8 ESCs were grown on 0.2% gelatin-coated plates without irradiated MEFs. The ESC medium was prepared by supplementing knockout Dulbecco’s Modified Eagle’s medium (Invitrogen) with 15% fetal bovine serum, 1 mM glutamax, 0.1 mM nonessential amino acids, 0.1 mM 2-mercaptoethanol, 1,000 units of LIF (ESGRO, ESG1106), 100 U ml -1 penicillin and 100 mg ml -1 streptomycin (Invitrogen). ESCs were treated with 10 μM SB431542 (Tocris Bioscience) for 2 or 48 h to inhibit TGF-beta signalling pathway [45] , [59] . Mouse ESC lines wild-type E14 (ola/129) and Eed -/- were grown on MEFs. Eed -/- ESCs were described previously [44] . In vitro differentiation of mouse ESCs For serum-free EB formation, ESCs were differentiated in defined culture system. EBs were formed by plating cells (1 × 10 5 cells ml -1 ) without LIF on Ultra Low Cluster Plate (Costar). ESCs were dissociated by TrypLE Express and cultured in serum-free defined media consisting of 75% Iscove’s modified Dulbecco’s medium and 25% Ham’s F12 media supplemented with 0.5 × of both N2 and B27 (without retinoic acid), 0.05% bovine serum albumin, 50 μg ml -1 ascorbic acid (Sigma) and 4.5 × 10 -4 M 1-thioglycerol as previously described [60] . After 2 days of EB formation, different dose (0, 5, 25 and 100 ng ml -1 ) of human Activin A (R&D systems) was added into the medium without dissociation/re-aggregation. At day 4, EBs were analysed by qPCR with reverse transcription and western blot analysis. For ChIP-seq, 100 ng ml -1 Activin (100 ng ml -1 ) or Activin (100 ng ml -1 ) plus SB431542 (10 μM) was added at EB day 2, and cultured for 2 days the for creation of day-4 EBs. Lentiviral-mediated RNA interference (RNAi) CGR8 ESCs were infected with lentivirus expressing control shRNA (no target: RHS 4750) or shHEB (RMM3981-97063804) with pLKO.1 construct (Open Biosystems). Lentiviral particles were generated by transfecting HEK293T cells with a pLKO.1 shRNA vector and packing vectors, psPAX2 and pMD2.G according to the RNAi consortium protocol [61] . For infection, mouse ESCs were incubated with lentiviral particles in ESC medium containing 8 μg ml -1 polybrene (Millipore). After 24 h, infection media were removed and replaced with ESC media with 1 μg ml -1 puromycin (Invitrogen). Puromycin-resistant colonies were analysed for knockdown of HEB from 6 days after infection (passage 2). RNA isolation, real-time PCR analysis To determine transcript levels in ESCs and differentiated cells, total RNA was extracted with RNeasy Kit (Qiagen) and complementary DNA (cDNA) was made from 1 μg using SuperScript III (Invitrogen) and random hexamers. For real-time PCR, we used the SYBR Green PCR master mix (Bio-Rad). The PCR was as follows: 95 °C for 5 min, 40 repeats with each repeat consisting of 95 °C for 30 s, 58 °C for 30 s, 72 °C for 30 s. This was followed by 72 °C for 7 min and a melt curve of 10-s cycles increasing by 0.5 °C from 55 °C to 95 °C. After data collection, melt curves were analysed visually to ensure that a single peak was present for each primer. Threshold amplification values (ct) were assigned by the iCycler analysis software (Bio-Rad). Housekeeping genes, beta-Actin (Actb) and Gapdh , served as internal controls. Relative gene expression was computed for each sample by comparing with control ESCs. PCR results were reported as mean±s.d. for three biological replicates. All primer sequences are listed in Supplementary Table 4 . 3SEQ analysis RNA-seq libraries were built using an approach which targets the 3′ end of each transcript (3SEQ) as described previously [62] . Three biological replicates from shControl or shHEB-targeted cells were prepared for each cell type: ESC and differentiated EB in the serum-free defined culture system, with or without Activin treatment. Total RNA was isolated using the RNeasy Plus Mini Kit (Qiagen) and then mRNA was purified using Dynabeads Oligo(dT) 25 (Invitrogen). The mRNA (400 ng) was heat sheared and reverse transcribed with a custom P7 oligo(dT)_Index primer containing Illumina-compatible adaptor sequence. cDNA fragments were end repaired and ligated to double-stranded P5 linker. The linker-ligated cDNA was size-selected for 200–350 bp fragments by 3% Nusieve agarose gels (Lonza) and amplified for 15 cycles. The quality of second size-selected library was assessed using the 2100 Bioanalyzer (Agilent) and Qubit (Invitrogen), and sequenced on the Illumina HiSeq 2000. Read sequences were trimmed to remove the 3SEQ adaptors and leading or trailing low-quality bases using Trimmomatic 0.32 with parameters ILLUMINACLIP 2:30:5, LEADING:3, TRAILING:3. Trimmed reads were aligned by STAR 2.3.0e (ref. 63 ) to the mm9 reference genome and a reference transcriptome prepared by combining Ensembl gene annotations with ENCODE RNA-seq data from E14 mouse ESCs using Cufflinks 2.2.1 (ref. 64 ); candidate splice junctions that were both non-canonical and unannotated were discarded. Reads with posterior probability of alignment ≥0.9 (MAPQ ≥10) were counted in the last 1 kb of each transcript by the featureCounts tool in Subread 1.4.5 (ref. 65 ). Transcript read counts were tested for significant differences between shHEB and shControl by DESeq2 1.2.8 (ref. 66 ), analysing each cell per treatment group independently; transcripts with no reads from any library were ignored. Immunoprecipitation and western blot analysis Cells were collected in lysis buffer (50 mM Tris pH 8.0, 150 mM NaCl, 1% NP-40) supplemented with a cocktail of protease inhibitors (Roche). Nuclear and cytoplasmic extracts were prepared using NE-PER Nuclear and Cytoplasmic Reagents (Pierce) according to the manufacturer’s protocol. For co-immunoprecipitation (coIP), 3 μg each antibody (SMAD2/3, sc-8332X, 2 μg μl -1 ; HEB, sc-357X, 2 μg μl -1 ; E2A, sc-349X, 2 μg μl -1 ) or rabbit IgG (1 μg μl -1 , R&D Systems) coupled with 20 μl Protein A beads (Invitrogen) was incubated overnight at 4 °C. Beads were washed four times with lysis buffer and eluted with SDS-loading buffer. Proteins were separated on SDS polyacrylamide gels, transferred onto polyvinylidene difluoride membranes (Amersham) and detected through horseradish-peroxidase conjugated secondary antibodies (Santa Cruz Biotechnology) and chemiluminescent ECL (Amersham). The primary antibodies used were anti-GATA4 (AF2606, 1:5,000) and SOX17 (AF1924, 1:5,000) from R&D Systems, anti-SMAD2/3 (sc-8332X, 1:6,000), HEB (rabbit antibody, sc-357X, 1:3,000; mouse antibody, sc-28365, 1:1,000), E2A (sc-349X, 1:2,000) and OCT4 (sc-5279, 1:3,000) from Santa Cruz Biotechnology, anti-LEFTY (ab22569, 1:5,000), TUBULIN (ab80779, 1:5,000), H3 Histone (1:5,000) and H3K4me3 (ab8580, 1:5,000) from Abcam and anti-EZH2 (1:2,000) from BD Biosciences. ChIP and ChIP-qPCR ChIP from mouse ESCs and differentiated ME was performed according to our previous report [32] using 100 μg of chromatin per IP. Briefly, cells were chemically crosslinked with 1% formaldehyde for 15 min at room temperature and the reaction was stopped by adding glycine (to 125 mM) for 5 min. The cells were rinsed with PBS and resuspended in lysis buffer (50 mM Tris pH8.1, 10 mM EDTA, 1% SDS) with protease inhibitor cocktail (Roche), and fragmented with a Branson 450 Sonifier (ten pulses at 60%) to a size range of 200 to 500 bp. Solubilized chromatin was diluted twofold in ChIP dilution buffer and, after removal of a control aliquot, immunoprecipitated with Protein A or G magnetic beads (Invitrogen) coupled with 5 μg of each antibody at 4 °C overnight. Immune complexes were washed sequentially with low salt immune complex wash, high salt immune complex wash, LiCl immune complex wash, and TE, and then eluted in elution buffer (1% SDS, 0.1 M NaHCO 3 ). The reverse crosslinking was performed at 65 °C overnight. After RNase A and Proteinase K treatment, sample was deproteinized with UltraPure Phenol: Chloroform: Isoamyl Alcohol (Invitrogen) and further purified with QIAquick PCR Purification Kit (Qiagen). The primary antibodies used for ChIP were anti-SMAD2/3 from R&D Systems, anti-HEB from Santa Cruz Biotechnology, anti-JARID2 from Novus Biologicals, anti-SUZ12 from Active Motif, anti-EED from Millipore and H3K27me3 from Upstate. DNA levels were first normalized to the internal control region in the first intron of Actb . Intergenic region in chromosome 8 (72,806,101–72,806,240) was also used for negative control for DNA binding [7] . Relative enrichment was calculated by dividing the normalized level of ChIPed DNA to that of input DNA at the corresponding locus. ChIP-qPCR results were reported as mean±s.d. for three ChIP biological replicates. Primers used for qPCR to quantify the ChIP-enriched DNA are listed in Supplementary Table 5 . ChIP-seq data analysis ChIP-seq libraries were prepared according to Illumina protocols and sequenced using Illumina Genome Analyzer; 36 base pair(bp) long reads were obtained. All sequences, including those for SUZ12, EZH2 and JARID2 (ref. 35 ), were mapped to the mouse reference genome (mm9) using ELAND software (Illumina Inc) and peaks called using QuEST 2.4 (ref. 67 ) in the DNAnexus platform ( https://dnanexus.com ) using a ‘transcription factor’ setting (bandwidth of 30 bp, regions size of 300 bp) and 25- or 30-fold ChIP to input enrichment for seeding the regions at <0.001 false discovery rate (FDR). For the enhancer marks comparison with HEB/SMAD2/3 elements in ESCs, we used the previously published ChIP-seq data for H3K27ac, H3K4me1 and p300 (ref. 38 ). Two replicates of histone marks, H3K27ac and H3K4me1, were combined and mapped to the mouse reference genome (mm9) using the DNAnexus platform, and performed peakcalling with ‘histone’ setting (bandwidth of 100 bp, regions size of 1,000 bp) and 15-fold ChIP to input enrichment for seeding the regions at <0.001 FDR. Two replicates of P300 were combined and mapped to mm9 and performed peakcalling with ‘transcription factor’ setting and 25-fold ChIP to input enrichment for seeding the regions at <0.001 FDR. We associated genes for each peak and the nearest genes within 100, 50 and 10 kb from the TSS as shown in the Supplementary Table 1 . We merged overlapping bound regions (minimum overlap 1 bp) using Galaxy ( http://main.g2.bx.psu.edu ), and analysis of GO enrichment for each data set was performed using GREAT (mm9, default settings, genome-wide background, http://great.stanford.edu ) [34] or DAVID v6.7 for the ‘Official Gene Symbol’ ( http://david.abcc.ncifcrf.gov ) and the significance was shown as Binom raw P -value for GREAT and EASE Score, a modified Fisher exact P -value, for DAVID. Gene expression comparison Aligned RNA-seq reads from ref. 43 were quantified for transcript abundances at known genes from the UCSC database [68] , as fragments per kilobase (kb) of transcript per million mapped reads by Cufflinks 2.1.1 with default parameters [64] . The difference in transcript abundance between mouse ESCs (ESC, untreated) and Activin-treated differentiated cells (ME, mesoderm and endoderm) samples was tested for statistical significance by Cuffdiff2 with default parameters (ibid.). For visualization and comparison, the log 10 of each gene’s P -value was signed by the direction of the difference between samples. The significance of the average increase in signed log 10 P -values between groups of genes was then computed with Welch’s one-sided two-sample t -test, with the ‘ESC and ME’ and ‘ME only’ groups pooled for comparison with the ‘ESC only’ group. Multifactorial comparison of ChIP-seq samples To measure the effects of differentiation and SB431542 treatment on HEB occupancy, we used UniPeak 1.0 (ref. 48 ) to combine all ChIP-seq data generated by this study (HEB in ESC and ME, with or without SB431542 treatment) into a single set of genome regions with enriched protein occupancy. We then selected only the HEB experiments and normalized the read counts in these regions with the regularized log transformation in DESeq2 version 1.2.1 (ref. 69 ). Accession codes. The ChIP-seq and 3SEQ data has been deposited in GEO under accession number GSE60286 . How to cite this article: Yoon, S.-J. et al. HEB associates with PRC2 and SMAD2/3 to regulate developmental fates. Nat. Commun. 6:6546 doi: 10.1038/ncomms7546 (2015).